Three types of genes underlying theGametophyte factor1locus cause unilateral cross incompatibility in maize Unilateral cross incompatibility (UCI) occurs between popcorn and dent corn, and represents a critical step towards speciation. It has been reported that ZmGa1P , encoding a pectin methylesterase ( PME ), is a male determinant of the Ga1 locus. However, the female determinant and the genetic relationship between male and female determinants at this locus are unclear. Here, we report three different types, a total of seven linked genes underlying the Ga1 locus, which control UCI phenotype by independently affecting pollen tube growth in both antagonistic and synergistic manners. These include five pollen-expressed PME genes ( ZmGa1Ps-m ), a silk-expressed PME gene ( ZmPME3 ), and another silk-expressed gene ( ZmPRP3 ), encoding a pathogenesis-related (PR) proteins. ZmGa1Ps-m confer pollen compatibility. Presence of ZmPME3 causes silk to reject incompatible pollen. ZmPRP3 promotes incompatibility pollen tube growth and thereby breaks the blocking effect of ZmPME3 . In addition, evolutionary genomics analyses suggest that the divergence of the Ga1 locus existed before maize domestication and continued during breeding improvement. The knowledge gained here deepen our understanding of the complex regulation of cross incompatibility. Reproductive isolation is one of the major driving forces of speciation and evolution [1] , [2] , and is generally classified as either prezygotic or postzygotic [3] . The nature of reproductive isolation in angiosperms involves multiple aspects, including pollen recognition, pollen tube growth, pollen tube reception and the fusion between male and female gametes [4] , [5] , [6] . Unilateral cross incompatibility (UCI) is a type of prezygotic reproductive isolation that occurs in maize between popcorn and dent corn varieties. Since it first description in 1902 [7] , a linked locus named Gametophyte factor1 ( Ga1 ) has been reported on the short arm of chromosome 4 [8] , [9] . It was further reported that the Ga1 locus is composed of three different haplotypes, Ga1-S, Ga1-M , and ga1 . Popcorn possesses the Ga1-S haplotype, and dent corn possesses the ga1 haplotype. ga1 plants accept any type of maize pollen; Ga1-S plants cannot be pollinated by ga1 pollen, but can pollinate all other genotypes; while Ga1-M plants exhibit wide compatibility in either corn type [10] . Previous studies have demonstrated that UCI is caused by failed growth of ga1 pollen tubes. After successful germination, ga1 pollen tubes arrest growth before reaching the ovules in Ga1-S silks [11] . Efforts to genetically dissect the Ga1 locus revealed that UCI is governed by at least two determinants: (i) a male determinant acting in pollen/pollen tubes and endows pollen tubes to become compatible for any type of silks. (ii) a female determinant acting in silk, enabling silk to reject pollen tubes that lack male determinant (incompatibility) [12] , [13] . Recently, ZmGa1P , encoding a pectin methylesterase, which is highly expressed in Ga1-S and Ga1-M pollen, has been shown as a male determinant of the Ga1 locus [14] . Moreover, ZmPME3 , was identified and shown to be highly expressed in Ga1-S but barely in ga1 silks [15] . It shares high similarity with Tcb1-f , a gene identified in teosinte and proved to be responsible for blocking maize pollen tubes [16] . Therefore, ZmPME3 was suggested as a likely candidate for the female determinant. However, how the female determinant functions, and the genetic relationship between male and female determinants at the Ga1 locus [17] , [18] , [19] still remained elusive. In this study, we use genetic analysis to separate the Ga1 locus into two functional components and identify seven causal genes, encoding three types of proteins. Transgenic approaches confirm that the seven genes harbor both male and female determinant functions, and work together to constitute the UCI system. Moreover, the three types of genes exhibit clear variation between cultivated, landrace and wild maize and thus provides an excellent system to deeply understand the history of maize domestication and improvement. The Ga1 locus contains two functional components To confirm that UCI in our genetic material is caused by abnormal pollen tube growth [8] , [15] , rather than failed gamete fusion (Fig. 1a ), we collected SK ( Ga1-S ) silks pollinated by Zheng58 (Z58, ga1 ) pollen and self-pollinated SK silks at 8 h and 24 h after pollination, respectively. We observed that Z58 pollen tubes were significantly shorter than those of SK pollen tubes in SK silks [2.07 ± 0.27 cm vs. 3.80 ± 0.34 cm ( P = 3.91E-15) at 8 h; 3.55 ± 0.72 cm vs. 12.49 ± 0.86 cm ( P = 9.90E-25) at 24 h)] (Supplementary Fig. 1a, b ). All observed SK pollen tubes were equivalent in length to the SK silks, By contrast, the longest pollen tubes of Z58 reached only about 30% of the total length of SK silks at 24 h after pollination, with a heavy callose deposition at the tip and arrest growth before reaching the ovule [11] [28 ± 5% vs. 100% ( P = 4.35E-30)] (Supplementary Fig. 1c, d ). When SK silks were cut shorter than 5 cm, we were able to harvest a few kernels pollinated by Z58 (Supplementary Fig. 1e ), implying that UCI is caused by abnormal Z58 pollen tube elongation rather than failed gamete fusion. This observation strongly suggests that promoting pollen tube growth is the key to overcome incompatibility. Fig. 1: Fine mapping and genomic structure of the Ga1 locus in maize. a The UCI phenotype: self-pollinated SK ( Ga1-S ), Zheng58 (Z58, ga1 ) and reciprocal crosses between SK and Z58. Scale bar = 2 cm. b Ga1 was fine mapped to a 2 Mb interval, flanked by markers M4 and M9. It contains two functional components, Component1 (M4-M7) and Component2 (M7-M9). SK represents the SK genotype, Z58 represents Zheng58 genotype and H represents heterozygous genotype. The numbers in each row represent the number of individuals in the progeny generated after self-fertilization of recombinant plants with the genotype on the left. P value represents the significance of the chi-square test. c Sequence alignment of the Ga1 locus between B73 and SK genomes. Syntenic blocks are highlighted by gray lines. Five ZmGa1Ps-m genes, one silk-expressed gene ZmPME3 , and four silk-expressed CRP genes are highlighted by green and orange boxes. Alignments of homologous genes on the B73 and SK genome are indicated by green and orange lines. Present-absent variations are indicated by gray dotted lines and absent genes are indicated by dotted boxes. d Gene structure alignment of ZmGa1Ps-m genes, silk-expressed gene ZmPME3 and ZmPRP3 compared between SK ( Ga1-S ), P178 ( Ga1-M ) and B73 ( ga1 ). The complete pectin methylesterase domains in ZmPME3 SK genes are highlighted in green. The incomplete pectin methylesterase domains in ZmPME3 P178 that is interrupted by a 2 bp insertion is highlighted in orange. Absent ZmPME3 B73 is indicated by orange dotted boxes. The complete pectin methylesterase domains in ZmGa1Ps-m SK and ZmGa1Ps-m P178 are highlighted in green. The incomplete pectin methylesterase domain in ZmGa1Ps-m B73 that due to a nonsense point mutation from G to A is highlighted in orange. The barwin domains in ZmPRP3 P178 and ZmPRP3 B73 are highlighted in orange boxes. Absent ZmPRP3 SK is indicated by green dotted boxes. White boxes represent coding sequence. UTR region is highlighted with gray boxes. e Expression patterns of thirteen PME genes, ZmPRP3 , Zm00001d048948 , Zm00001d048949 , and Zm00001d048950 in silk and pollen of SK ( Ga1-S ), P178 ( Ga1-M ) and Z58 ( ga1 ) as determined by RNA-seq data. TPM, Transcripts Per kilobase per Million mapped reads. “*” highlight with red presents non-functional transcript of ZmPME3 in Ga1-M silk. Full size image Next, a Recombination Inbred Line (RIL) population between Z58 × SK was developed, and genotyped using high-density markers [20] , [21] . We detected a segregation distortion locus that the genotypes of two parents are significantly deviating from the expected ratio (1:1) on chromosome 4 from 2 Mb to 25 Mb (Supplementary Fig. 2 ), which overlapped with the defined the Ga1 locus in previous reports [8] , [22] , [23] , [24] . Approximately 4900 individuals from the Z58 × SK F 2 population were subjected to fine map the Ga1 locus using genotypic segregation distortion as a phenotype. Fine mapping results revealed that the Ga1 locus can be separated into two components that both influenced segregation distortion, we named here as Component1 (between marker M4 and M7) and Component2 (between marker M7 and M9) (Fig. 1b and Supplementary Fig. 3 ). When individuals possessed the SK genotype at Component1, segregation distortion completely disappeared (R5, P = 0.46, n = 197; Fig. 1b ), suggesting that Component1 is a major locus for overcoming cross incompatibility. Component2 affected the degree of segregation distortion only if Component1 was heterozygous. When Component2 was homozygous for the SK genotype, Component1 showed the strongest segregation distortion (R2, P = 2.66E-17, n = 164, Fig. 1b ). When Component2 was heterozygous, Component1 showed lighter segregation distortion (R1, P = 7.25E-06, n = 230; R4, P = 6.90-08, n = 289, Fig. 1b ). When Component2 was homozygous for the Z58 genotype, Component1 did not show segregation distortion (R3, P = 0.64, n = 199, Fig. 1b ). To further confirm function of the two components, we used a diverse Association Mapping Panel (AMP) [25] as male parents to pollinate CML304 ( Ga1-S ), and took the CML304 seed set ratio as a phenotype for a genome-wide association study (GWAS) [26] (see Materials and Methods for details). SNPs significantly associated with seed set ratio were identified within the Component1 region (Supplementary Fig. 4 ). These results demonstrated that Component1 contains a male determinant that enables pollen tubes to overcome the block effect of Ga1-S silks, and that the function of Component2 depends on Component1. Component2 is most likely being a weak regulator affecting UCI. Genomic structure analysis and identification of candidate genes at the Ga1 locus Traditional fine mapping to clone the Ga1 locus has been pursued for years, the interval cannot be further narrowed below 1.7 Mb, suggesting that huge structural variations between the Ga1-S and ga1 genomes may not allow genetic mapping. A high-quality SK genome has recently become publicly available [27] . Although the Z58 genome is still not available, B73 ( ga1 ) shows the same UCI phenotype as Z58. We were thus able to compare the genomic sequences of the Ga1 locus between B73 [28] and SK. Despite a similar size of the Ga1 locus in the B73 and SK genomes, a very different sequence, with few syntenic blocks between markers M4 and M7 was detected (Fig. 1c and Supplementary Fig. 4e ). This explains why it was so difficult to find sufficient recombinant individuals for fine mapping strategies. In the region of Component1, 28 genes were annotated within the SK genome. These include 13 consecutive PECTIN METHYLESTERASE ( PME ) genes (Supplementary Data 1 ). However, in the corresponding Component1 region of B73, there is only one annotated gene, Zm00001d048936 , (also known as the ga1 type ZmGa1P ), highly expressed in pollen and exhibiting synteny to the PME gene cluster (Fig. 1c, d and Supplementary Data 2 ). RNA-seq data from nine SK tissues further confirmed that five of the thirteen PME genes are highly expressed in SK pollen ( ZmGa1Ps-m : ZmGa1P.1, ZmGa1P.2, ZmGa1P.3, ZmGa1P.4 , and ZmGa1P.5 ), and one gene ( ZmPME3 ) is highly expressed in SK silks (Supplementary Fig. 5 ). A pollen-expressed PME gene at the Ga1 locus, ZmGa1P , was found in SDGa25 ( Ga1-S ) and previously reported to be responsible for cross incompatibility by controlling the equilibrium of pectin esterification / de-esterification at the apical region of the growing pollen tube [14] , [29] . We found that ZmGa1Ps-m genes not only exhibit high sequence identity to one another (identity > 95%), but also to ZmGa1P (identity > 95%), with only a few single nucleotide polymorphisms (SNPs) (Supplementary Fig. 6 ). Most of these cause synonymous mutations (Supplementary Fig. 7 ). When comparing ZmGa1Ps-m genes with Zm00001d048936 , which has been proved as a non-functional homologous gene of ZmGa1P in the B73 genome, we found that Zm00001d048936 ( ga1 ) harbors a nonsense point mutation from G to A (Supplementary Fig. 8 ), producing premature termination (Supplementary Fig. 9 ), consisting with previous findings [14] . To further ascertain if ZmGa1Ps-m genes contribute to regulating pollen tube growth, we extracted RNA from pollen of SK ( Ga1-S ), P178 ( Ga1-M ) and Z58 ( ga1 ) and determined the expression level of the PME gene cluster (Supplementary Data 3 ). SNPs in the RNA-seq data clearly distinguished ZmGa1Ps-m genes from each other (Supplementary Figs. 10 and 11 ) and revealed their respective high expression in SK and P178 pollen, but were absent in Z58 pollen (Fig. 1e and Supplementary Fig. 12 ). This finding indicates that all ZmGa1Ps-m genes are unique genes, likely required to overcome the Ga1-S barriers. Moreover, sequence alignment between SK and B73 revealed that ~800 bp coding sequence of the each ZmGa1Ps-m genes was missing across the entire B73 genome. A similar result was also observed in the HP301( Ga1-S ) genome [30] (Supplementary Fig. 13 ), indicating a presence-absence variation (PAV) [31] . Based on the CML304 ( Ga1-S ) seed set ratios crossed with AMP pollen, and the seed set ratios from crosses by using AMP lines each as a female parent and Z58 ( ga1 ) as a male parent, AMP inbred lines could be divided into three haplotypes (see Materials and Methods for details): ga1 ( n = 303), Ga1-M ( n = 82), and Ga1-S ( n = 7). After counting mapped reads from AMP whole genome re-sequencing data [27] , we found that ZmGa1Ps-m genes were absent in all ga1 but present in Ga1-M and Ga1-S lines. This demonstrated that PAV of ZmGa1Ps-m genes is widespread at the population level (Supplementary Fig. 14 ). Therefore, we assumed that there are also multiple copies of ZmGa1P in the SDG25a genome. However, limited by the length of the BAC clone, it is hard to assemble all the peptide fragment from multiple highly similar ZmGa1P genes in an interval close to 1.5 Mb. Silk-expressed ZmPME3 has been reported as a candidate female gene involved in UCI [15] . We also observed that ZmPME3 is the only PME gene within the Component1 region and that it is highly expressed in SK silks (Fig. 1e and Supplementary Fig. 5 ), but absent from the entire B73 genome (Fig. 1c, d ). However, previous studies also pointed out that ZmPME3 has a frame-shift mutation in some Ga1-M lines, while a few lines possess intact ZmPME3 transcripts [15] , [32] , which makes it difficult to conclude whether ZmPME3 harbors female determinant function. In our next investigation, we extracted RNA from silk of SK ( Ga1-S ), P178 ( Ga1-M ), Z58 ( ga1 ) and 70 selected inbred lines from the AMP, containing ga1 ( n = 34), Ga1-M ( n = 30) and Ga1-S ( n = 6) haplotypes. Both RNA-seq (Supplementary Data 4 ) and quantitative RT-PCR analysis (Supplementary Data 5 ) confirmed that ZmPME3 is expressed in silks of all selected Ga1-S and a proportion of Ga1-M lines, but conversely is not expressed in any silks of ga1 lines (Fig. 1e and Supplementary Fig. 15a ). Sequencing of ZmPME3 transcripts from selected Ga1-M and Ga1-S silks implied that the coding sequences derived from Ga1-M silks is interrupted by a 1 or 2 bp insertion (Supplementary Fig. 15b ), which is consistent with the previous study [15] . It thus appears that ZmPME3 generates functional transcripts with abundant expression in all Ga1-S lines, which makes ZmPME3 at least consider as a candidate female determinant of the Ga1-S type, enabling Ga1-S silks to block ga1 pollen tube growth. We next analyzed expression levels of the annotated genes in the Component2 region using pollen and silks of SK ( Ga1-S ), P178 ( Ga1-M ) and Z58 ( ga1 ). Notably, this region contains four genes, encoding cystein-rich proteins ( CRPs ) [33] , [34] . One of them, Zm00001d048947 , which encodes a small protein containing a barwin domain (known as Zea mays pathogeneesis-related protein3 ZmPRP3 [35] ), is absent from the entire SK genome (Fig. 1d ), but is highly expressed in Z58 and P178 silks (Fig. 1e and Supplementary Fig. 16 ). Moreover, 20 × re-sequencing data of inbred lines from AMP further confirmed that ZmPRP3 is absent from all Ga1-S lines, but present in 90% of Ga1-M lines and 99% of ga1 lines (Supplementary Fig. 17 ). Quantitative RT-PCR results (Supplementary Fig. 15a ) further showed that ZmPRP3 is expressed in all tested ga1 and Ga1-M lines, and contains a highly conserved peptide sequence with five cysteines (Supplementary Fig. 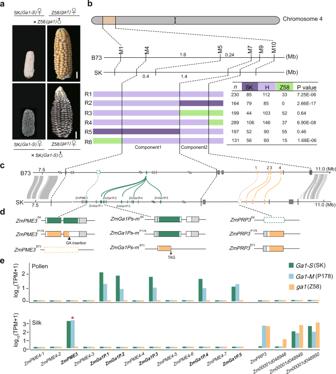Fig. 1: Fine mapping and genomic structure of theGa1locus in maize. aThe UCI phenotype: self-pollinated SK (Ga1-S), Zheng58 (Z58,ga1) and reciprocal crosses between SK and Z58. Scale bar = 2 cm.bGa1was fine mapped to a 2 Mb interval, flanked by markers M4 and M9. It contains two functional components, Component1 (M4-M7) and Component2 (M7-M9). SK represents the SK genotype, Z58 represents Zheng58 genotype and H represents heterozygous genotype. The numbers in each row represent the number of individuals in the progeny generated after self-fertilization of recombinant plants with the genotype on the left.Pvalue represents the significance of the chi-square test.cSequence alignment of theGa1locus between B73 and SK genomes. Syntenic blocks are highlighted by gray lines. FiveZmGa1Ps-mgenes, one silk-expressed geneZmPME3, and four silk-expressedCRPgenes are highlighted by green and orange boxes. Alignments of homologous genes on the B73 and SK genome are indicated by green and orange lines. Present-absent variations are indicated by gray dotted lines and absent genes are indicated by dotted boxes.dGene structure alignment ofZmGa1Ps-mgenes, silk-expressed geneZmPME3andZmPRP3compared between SK (Ga1-S), P178 (Ga1-M) and B73 (ga1). The complete pectin methylesterase domains inZmPME3SKgenes are highlighted in green. The incomplete pectin methylesterase domains inZmPME3P178that is interrupted by a 2 bp insertion is highlighted in orange. AbsentZmPME3B73is indicated by orange dotted boxes. The complete pectin methylesterase domains inZmGa1Ps-mSKandZmGa1Ps-mP178are highlighted in green. The incomplete pectin methylesterase domain inZmGa1Ps-mB73that due to a nonsense point mutation from G to A is highlighted in orange. The barwin domains inZmPRP3P178andZmPRP3B73are highlighted in orange boxes. AbsentZmPRP3SKis indicated by green dotted boxes. White boxes represent coding sequence. UTR region is highlighted with gray boxes.eExpression patterns of thirteenPMEgenes,ZmPRP3,Zm00001d048948,Zm00001d048949, andZm00001d048950in silk and pollen of SK (Ga1-S), P178 (Ga1-M) and Z58 (ga1) as determined by RNA-seq data. TPM, Transcripts Per kilobase per Million mapped reads. “*” highlight with red presents non-functional transcript ofZmPME3inGa1-Msilk. 18 and Supplementary Table 1 ). Considering the key roles of CRPs in plant defense and reproduction [36] , [37] , [38] , we thus speculated that ZmPRP3 may serve as a positive regulator to accelerate pollen tube growth in ga1 and Ga1-M silks, The other three CRP genes ( Zm00001d048948, Zm00001d048949 , and Zm00001d048950 ) display high sequence similarity (identity > 80%) to ZmPRP3 (Supplementary Fig. 19 ), but exhibit different expression pattern (Fig. 1e ). While Zm00001d048948 is only expressed in ga1 silks, Zm00001d048949 and Zm00001d048950 are expressed in all genotypes, we thus considered only ZmPRP3 to be the best candidate of a causal gene of Component2. Transgenic experiments support the causal roles of identified ZmGa1Ps-m , ZmPME3 , and ZmPRP3 in regulating pollen tube growth To verify whether ZmGa1Ps-m genes all regulate pollen tube growth, we over expressed each ZmGa1Ps-m gene individually using the ubiquitin promoter in the KN5585 ( ga1 ) background [39] . However, PME gene expression level in the transgenic over-expression lines reached 2% to 13% of that found in SK pollen (Fig. 2a ), which is lower than that of ZmGa1P in B104 ( ga1 ) pollen (a 6287 bp genomic fragment containing ZmGa1P and its native promoter was cloned from SDGa25 and introduced into the inbred line B104 to verify ZmGa1P function) [14] . We speculate this discrepancy is caused because the ubiquitin promoter is weaker in pollen compared with the ZmGa1P promoter. At 8 h after pollination, the maximal length of pollen tubes that over-expressed ZmGa1Ps-m genes were significantly longer than those of the wild type [WT, KN5585 ( ga1) ] in SK silks, ranging from 1.46 times longer for ZmGa1P.4 [1.69 ± 0.19 cm vs. 1.15 ± 0.29 cm ( P = 2.40E-08)] to 1.81 times longer for ZmGa1P.5 [2.08 ± 0.31 cm vs. 1.15 ± 0.29 cm ( P < 2.00E-16)]. However, they only reached 44.5–54.7% of the length of SK pollen tubes [ ZmGa1P.4 , 1.69 ± 0.19 cm vs. 3.92 ± 0.41 cm ( P < 2.00E-16); ZmGa1P.5 , 2.08 ± 0.31 cm vs. 3.92 ± 0.41 cm ( P < 2.00E-16)] (Fig. 2b ). In summary, there is a clear positive correlation between pollen tube length and ZmGa1Ps-m genes expression levels. As a consequence, SK plants fertilized with pollen from transgenic lines over-expressing ZmGa1P.2 exhibited a significant increase in seed number compared with WT pollen [12.6 ± 7% vs. 0.00 ( P = 0.0043)] (Fig. 2c , and Supplementary Fig. 20 ). These data together indicate that ZmGa1Ps-m are causal genes, and that their accumulative expression level accelerate Ga1-S and Ga1-M pollen tube growth, which ultimately lead pollen tubes to overcome the Ga1-S barrier. Fig. 2: Transgenic confirmation that ZmGa1Ps-m , Zm PME3 and ZmPRP3 regulate pollen tube growth. a Quantitative expression analysis of ZmGa1Ps-m genes in pollen of over-expressed transgenic plants, WT [KN5585 ( ga1 )] and SK. b Comparison of the longest pollen tubes in SK silks at 8 h after pollination, using pollen of WT, SK, and over-expressed lines for each ZmGa1Ps-m genes. c Statistical analysis of SK seed set ratio crossed with SK, WT, ZmGa1P.2 over expressed lines pollen . d Quantitative expression analysis of ZmPME3 in silks of ZmPME3 over expressed lines, WT and SK. #1-#3 represents three ZmPME3 over expressed transgenic plants. #4-#7 represents four ZmPME3 over expressed transgenic plants. e Comparison of the longest pollen tubes of WT [KN5585 ( ga1 )] at 8 h after pollination in silks of ZmPME3 over expressed, WT and SK plants. f Statistical analysis of the seed set ratio from crosses by using SK, WT, and ZmPME3 over expressed plants each as a female parent and WT [KN5585 ( ga1 )] as a common male parent. g Sequence of ZmPRP3 in WT and CRISPR-Cas9 edited plants. Lines in blue denote the sgRNA, and the protospacer-adjacent motif (PAM, NGG) is indicated by the black square. White box indicates the coding sequence and barwin is highlighted with brown boxes. h Comparison of the longest pollen tubes of WT [KN5585 ( ga1 )] at 8 h after pollination in silks of WT and CR-Zmprp3 plants. i Comparison of the longest pollen tubes of SK at 8 h after pollination in silks of WT and CR-Zmprp3 plants. j Statistical analysis of seed set ratio from crosses by using CR-Zmprp3 and WT each as a female parent and WT [KN5585 ( ga1 )] as a common male parent. For a – f , data were analyzed according to the LSD test. For h – j , data were analyzed by two-tailed Student’s t -test. Error bars represent mean + SD ( a – e , h , i ). a, b, c indicate significant differences ( P < 0.01) ( a – f ). Asterisks indicate significant differences (** P < 0.01) ( h ), ns (not significant, P > 0.05) ( j ). Relative expression ( n = 3, biologically independent samples) ( a , d ). Longest pollen tube length or harvest kernel number ( n = number of biologically independent samples in each column) ( b , c , e ). In box plots, the center line represents the median, box edges delimit lower and upper quartiles and whiskers show the highest and lowest data points, n present sample size ( f , j ). Source data are provided as a Source Data file. Full size image We also over-expressed ZmPME3 transcript derived from the SK genome in the KN5585 background to investigate whether ZmPME3 is capable of blocking ga1 pollen tube growth. Although transgenic plants maintained a lower ZmPME3 expression levels in silks than SK (reaching only about 2 ~ 10% of the SK level), they expressed far more ZmPME3 transcripts than WT [KN5585 ( ga1) ]. This led to a slower KN5585 ( ga1 ) pollen tube growth rate in silks of three over-expressed ZmPME3 plants, at 8 h after pollination [2.17 ± 0.38 cm, 2.04 ± 0.42 cm and 2.14 ± 0.42 cm vs. 4.17 ± 0.23 cm ( P < 2.00E-16)]. However, the longest KN5585 ( ga1 ) pollen tubes in silks of over-expressed ZmPME3 plants were still nearly two times longer than those in SK silks [2.17 ± 0.38 cm, 2.04 ± 0.42 cm and 2.14 ± 0.42 cm vs. 1.15 ± 0.29 cm ( P = 8.30E-13; P = 8.30E-12; P = 8.30E-15)] (Fig. 2d, e ). This suggests that ZmPME3 is a causal female determinant gene of UCI in the Component1 region, conferring silks to reject ga1 pollen. Its expression level is negatively related to the growth rate of ga1 pollen tubes. Notably, we observed that KN5585 ( ga1) pollen crossed onto ZmPME3 OE+ lines resulted in full seed set (Fig. 2f and Supplementary Fig. 20 ). This may be due to insufficient expression of ZmPME3 in silks, or there are other factors that exist in ga1 silks and rescue the cross incompatibility phenotype. To further investigate the roles of ZmPRP3 identified in the Component2 region in regulating pollen tube growth, ZmPRP3 and its three homologs were each knocked out by CRISPR/Cas9 in KN5585 inbred lines to yield the corresponding homozygous null mutants, referred to here as CR-Zmprp3, CR-Zm00001d048948, CR-Zm00001d048949 and CR-Zm00001d048950 . Genome sequencing identified a 147 bp deletion in the first exon of ZmPRP3 (Fig. 2g ), resulting in a deletion of 49 amino acids that included the barwin domain. At 8 h after pollination, KN5585 ( ga1) pollen tubes grew significantly slower in the CR-Zmprp3 silks compared to WT [KN5585 ( ga1 )] silks [2.16 ± 0.29 cm vs. 4.18 ± 0.23 cm ( P = 1.51E-26)] (Fig. 2h ). With the exception of CR-Zmprp3 , none of the Zm00001d048948, Zm00001d048949 and Zm00001d048950 knock-out lines affected the KN5585 pollen tube growth rate (Supplementary Figs. 21 and 22 ). Furthermore, SK pollen tubes showed comparable growth rates in both CR-Zmprp3 and WT silks [3.71 ± 0.35 vs. 3.99 ± 0.33 ( P = 0.034)] (Fig. 2i ). We thus conclude that only ZmPRP3 contributes to regulating ga1 pollen tube growth, but it does not influence Ga1-S pollen tubes. KN5585 pollen crossed onto CR-Zmprp3 resulted in successful crosses (Fig. 2j and Supplementary Fig. 20 ), demonstrating that ZmPRP3 alone is not sufficient to regulate UCI. RNA-Seq analysis on silks of Recombination Lines (RL) and ZmPRP3 knock-out lines were next used to elucidate which pathway might be controlled by ZmPRP3 . 305 differentially expressed genes (DEGs) with fold change >2 were detected in lines expressing ZmPRP3 compared to those lacking ZmPRP3 . The DEGs were associated with 300 different Gene Ontology (GO) terms and the most enriched term was related to metal ion binding ( n = 55) (Supplementary Fig. 23 ). RNA-seq analysis in RL silks expressing ZmPME3 compared to those lacking ZmPME3 identified 10 DEGs, from which ZmPME3 itself exhibited the highest fold change (Supplementary Fig. 24 ). After comparing the two different groups of DEGs, we found that the absence of ZmPRP3 did not cause change in expression level of any PME genes. The degree of methylesterification (DM) of silk cell walls in ZmPME3 over-expression lines ( ZmPME3 OE+ ), ZmPRP3 knock-out lines ( CR-Zmprp3 ), SK and WT [KN5585 ( ga1 )] were also compared using LM20 and LM19, antibodies that preferentially recognizes methylesterified pectin [40] , [41] and low-methylesterified homogalacturonans (HGs) [42] respectively. SK and ZmPME3 OE+ silk cells exhibited weaker fluorescence intensity compared to the WT and CR-Zmprp3 using LM20 antibody (Supplementary Fig. 25 ). On the contrary, the fluorescence intensity of cells appeared stronger in CR-Zmprp3 and WT silks using LM19 antibody (Supplementary Fig. 26 ). These results indicated that the DM of cells in SK and ZmPME3 OE+ are lower than that of WT and CR-Zmprp3 . The fluorescence intensity of CR-Zmprp3 and WT silk cells have no difference under two conditions, suggesting ZmPRP3 does not affect the DM of silk cells. Altogether, this indicates that there exist additional mechanisms regulated by ZmPRP3 and differ from ZmPME3 activity, which also contribute to the regulation of UCI. Pollen and silk expressed ZmGa1Ps-m, ZmPME3 and ZmPRP3 constitute the UCI system in maize To further investigate the genetic relationship between silk-expressed ZmPRP3 and ZmPME3 and how they work together to regulate ga1 pollen tube growth, we observed Z58 pollen tube growth rates in silks of three recombinants: R2, R3, and R5 (Fig. 1b ). Quantitative RT-PCR analysis confirmed that the expression levels of ZmPME3 in silks were reduced by about half in heterozygous lines compared with homozygous lines for the SK genotype at Component1. ZmPRP3 is only expressed in lines in which Component2 harbors the Z58 genotype (Fig. 3a ). At 8 h after pollination, Z58 pollen tubes grew longer in silks of RL-Component1 Heterozygous -Component2 Z58 (R H-Z58 ) plants than in the RL-Component1 Heterozygous -Component2 SK (R H-SK ) plants [3.99 ± 0.43 cm vs. 2.49 ± 0.38 cm, ( P = 2.29E-22)] (Fig. 3b ). However, they showed a comparable growth rate in silks of RL-Component1 SK -Component2 SK (R SK-SK ) and RL-Component1 SK -Component2 Z58 (R SK-Z58 ) [2.07 ± 0.28 cm vs. 2.06 ± 0.26 cm, ( P = 0.93)] (Fig. 3b ). These results illustrate that the effect of Component2 on regulating pollen tube growth depends on Component1 genotype, is only relevant when Component1 is heterozygous. Component2 Z58 promotes Z58 pollen tube growth. This observation explains the lack of segregation distortion in R3 (Fig. 1b ). Fig. 3: Genetic relationship between three types of genes of the Ga1 locus. a Quantitative expression analysis of ZmPRP3 and ZmPME3 in silks of R SK-Z58 , R SK-SK , R H-Z58 , and R H-SK . b Comparison of the longest pollen tubes of Z58 at 8 h after pollination in silks of R SK-Z58 and R SK-SK silks, and in R H-Z58 and R H-SK . c Quantitative expression analysis of ZmPME3 in silks of WT, ZmPME3 OE+ , CR-Zmprp3 , and ZmPME3 OE+ / CR-Zmprp3 . #2 represents ZmPME3 OE+ plant. H1 and H2 represent two ZmPME3 OE+ / CR-Zmprp3 plants. d Comparison of the longest pollen tubes of WT [KN5585 ( ga1 )] at 8 h after pollination in silks of CR-Zmprp3 , ZmPME3 OE+ , WT, SK and ZmPME3 OE+ /CR-Zmprp3 plants. e Quantitative expression analysis of ZmPME3 in silks of CR-Zmprp3, ZmPME3 OE+ , WT, SK and ZmPME3 OE+ /CR-Zmprp3 plants. H3-H8 represents six ZmPME3 OE+ /CR-Zmprp3 plants. #4-#7 represents four ZmPME3 OE+ plant. f Statistical analysis of the seed set ratio from crosses by using SK, ZmPME3 OE+ , CR-Zmagp1 , ZmPME3 OE+ /CR-Zmagp1 and WT each as a female parent, WT [KN5585 ( ga1 )] as a common male parent. H3-H8 represents six ZmPME3 OE+ /CR-Zmprp3 plants. #4-#7 represent four ZmPME3 OE+ plants. g Crossing experiments showing ears of WT after self-pollination and crosses when SK, ZmPME3 OE+ , CR-Zmagp1 , ZmPME3 OE+ /CR-Zmagp1 were used as female parents, WT [(KN5585, ga1 )] pollen was used as male parent. Scale bar = 2 cm. h ga1 and Ga1-M s ilk-expressed ZmPRP3 acts as an accelerator, promoting the growth of ga1 pollen tubes. i Silk-expressed ZmPME3 exists in Ga1-S silk and is a female determinant that blocks ga1 pollen tube grow through silk. j ZmGa1Ps-m genes are male determinants, which exist in Ga1-S and Ga1-M pollen and can completely overcome block effect of ZmPME3 . k When ZmPME3 is heterozygous, introducing ZmPRP3 can effectively break the block effect of ZmPME3 , promote ga1 pollen tube growth. For a , c – f , data were analyzed according to the LSD test. For b , data were analyzed by two-tailed Student’s t -test. Error bars represent mean + SD ( a – e ). a, b, c indicate significant differences ( P < 0.01) ( a , c – f ). Asterisks indicate significant differences (** P < 0.01) ( b ). ns (not significant, P > 0.05) ( b ). Relative expression ( n = 3, biologically independent samples) ( a , c , e ). Longest pollen tube length ( n = number of biologically independent samples in each column) ( b , d ). In box plots, the center line represents the median, box edges delimit lower and upper quartiles and whiskers show the highest and lowest data points, n present sample size ( f ). Source data are provided as a Source Data file. Full size image To test whether the relationship between the two functional components depends on ZmPRP3 and ZmPME3 , we crossed CR-Zmprp3 cas9-positive plants with ZmPME3 over-expression plants. In the resultant hybrid plants, ZmPRP3 was edited and generated a 147 bp deletion ( ZmPME3 OE+ / CR-Zmprp3) (Figs. 2g and 3c ). At 8 h after pollination, we observed that the length of KN5585 ( ga1) pollen tubes went from longest to shortest as follows: in WT [KN5585 ( ga1 )] silks (4.18 ± 0.23 cm) > in CR-Zmprp3 (2.16 ± 0.29 cm) or in ZmPME3 OE+ (2.04 ± 0.42 cm) silks > in ZmPME3 OE+ / CR-Zmprp3 silks (1.22 ± 0.23 cm; 1.35 ± 0.20 cm) > in SK silks (1.15 ± 0.29 cm) (Fig. 3d ). Furthermore, the seed set ratios in crosses between ZmPME3 OE+ /CR-Zmprp3 and WT were significantly reduced and comparable to that of crosses between SK and WT. (Fig. 3e–g and Supplementary Fig. 20 ). Collectively, our results revealed that three types of genes possess both male and female determinant functions, independently regulate the growth rate of pollen tubes and thus affect cross incompatibility in maize. Based on the classic genetic model of the Ga1 locus [32] , we are now ultimately able to demonstrate causal genes governing the UCI system that balance antagonistic and synergistic effects. ZmGa1Ps-m genes are male determinants that are capable to endow Ga1-S and Ga1-M pollen with compatibility in any type of silks. Silk-expressed ZmPME3 is a female determinant that blocks ga1 pollen tube growth. On this basis, the silk-expressed gene ZmPRP3 that exists in ga1 and Ga1-M silks acts as an accelerator of pollen tube growth. Knocking out ZmPRP3 and over-expressing ZmPME3 produces the greatest effect on blocking ga1 pollen tube. Introducing ZmPRP3 in the heterozygous ZmPME3 background can effectively break the block effect of ZmPME3 , promote ga1 pollen tube growth (Fig. 3h–k and Supplementary Fig. 27 ). The presence of ZmPRP3 may explain why a few Ga1-M silks with intact ZmPME3 gene and ZmPME3 OE+ plants can still be fertilized by ga1 pollen as reported also in the previous study [15] . The Ga1 locus diverged before maize domestication and was further modified during maize improvement We next attempted to study the evolutionary origin of the Ga1 locus. For this purpose, we performed a principal component analysis (PCA) with 130,680 combined SNPs (53,173 SNPs derived from the B73 reference genome and 77,507 derived from the SK reference genome) around the Ga1 locus on 845 maize germplasms [392 diverse maize inbred lines, 336 landraces and 117 wild maize [ Z.mays ssp parviglumis ( n = 68), hereafter named parviglumis ; Zea mays ssp. mexicana ( n = 49),hereafter named mexicana ] [43] . PC1 clearly separated parviglumis and mexicana from maize (landrace, ga1 , Ga1-M, Ga1-S type lines), PC2 separated parviglumis into two sub-clusters [ par1 ( n = 19) and par2 ( n = 49)] (Fig. 4a ), as well as landraces [ lan1 ( n = 236) and lan2 ( n = 100)] and modern maize [ ga1 ( n = 303) and Ga1-S/Ga1-M ( n = 7/82)] (Fig. 4a ). Notably, mexicana is most closely related to par2, lan1 contained ga1 type lines, and lan2 contained Ga1-M and Ga1-S type lines. We next genotyped ZmGa1Ps-m and ZmPRP3 genes across all 820 lines by calculating mapped reads count, and found that ZmPRP3 was present in all lines except Ga1-S type lines (Supplementary Fig. 28 and Supplementary Data 6 ). ZmGa1Ps-m genes were present in both Ga1-M and Ga1-S , but not in ga1 type lines. Moreover, the mapped reads count of ZmGa1Ps-m genes in par1 were significantly higher than in par2 (Supplementary Data 6 ). Similar trends also appeared in the landrace (Supplementary Data 6 ) where ZmGa1Ps-m genes were almost absent in lan1 but displayed enriched mapped reads count in lan2 (Fig. 4b and Supplementary Fig. 28 ). The haplotype analysis on ZmPME3 further showed that par1 , lan1 and ga1 displayed a very consistent haplotype, while a proportion of par2, mexicana and lan2 possessing ZmPME3 haplotype that were more similar to Ga1-S and Ga1-M type lines (Supplementary Fig. 29 ). These results suggest that the origin of Ga1-S and Ga1-M type lines are close and related to par2, mexicana and lan2 . Fig. 4: Evolution and modification of the Ga1 locus during maize domestication. a Principal component analysis (PCA) of the Ga1 locus in parvivglumis , mexicana ( mex ), landraces, Ga1-M, Ga1-S and ga1 inbred lines. b Mapped reads count of ZmGa1P.1 in the two parviglumis subgroups ( par1, par2 ), mexicana (mex) , two landrace subgroups ( lan1, lan2 ) and modern maize subgroups ( Ga1-S, Ga1-M and ga1 inbred lines). ** P < 0.01 (two-tailed Student’s t -test and Wilcoxon ranked sum test). In box plots, the center line represents the median, box edges delimit lower and upper quartiles and whiskers show the highest and lowest data points. n present sample size. Mapped reads counts are provided in Supplementary Data 6 . c A putative evolutionary history of the Ga1 locus during domestication and improvement. The genotype of ZmGa1Ps-m is highlight with red, the genotype of ZmPME3 and ZmPRP3 are highlight with blue. −+ presents a haplotype that lost ZmGa1Ps-m and ZmPME3 (lack of complete gene sequences in the genome) but possesses ZmPRP3 . +++ presents a haplotype that possesses ZmGa1Ps-m , ZmPME3 (with potential enzymatic activity) and ZmPRP3. ++− presents a haplotype possesses ZmGa1Ps-m , functional ZmPME3 but lost ZmPRP3. +−+ presents a haplotype possesses ZmGa1Ps-m, ZmPRP3 but ZmPME3 lost their funtion (due to 1 or 2 bp insertion). d Eight cross combinations across three types of genes. ZmGa1Ps-m genes are highly expressed in pollen, the genotype of ZmGa1Ps-m is highlight with red. ZmPME3 and ZmPRP3 are expressed in silk, the genotype of ZmPME3 and ZmPRP3 are highlight with blue. Three haplotypes exist in modern maize inbred lines [ ga1 :−+; Ga1-S : + + −; Ga1-M : + − + ]. One haplotype exists in wild teosinte [ par2/Mexicana : +++]. Null haplotype presents cross incompatibility between ga1 pollen and Ga1-S silk [ ZmGa1Ps-m-, ZmPME3 + , ZmPRP3- (−+−)]. Three artificial haplotypes that do not exist in natural collections were: ga1 pollen crossed onto ZmPME3 over expressed lines [ ZmGa1Ps-m- , ZmPME3 + , ZmPRP3 + (−++)] Ga1-S pollen crossed onto ZmPRP3 knock-out lines [ ZmGa1Ps-m + , ZmPME3-, ZmPRP3- ( +− )], and ga1 pollen crossed onto ZmPRP3 knock-out lines [ ZmGa1Ps-m-, ZmPME3-, ZmPRP3- (−−−)], which all resulted in successful crosses, proving the three artificial haplotypes are fertile. The number labeled in black represent the proportion of male gametes, female gametes and zygote haplotype in AMP. Full size image Altogether, these results strongly indicated that the divergence of the Ga1 locus occurred already before maize was domesticated from teosinte, divergence continued during further maize improvement. One evolutionary branch ( par1 − lan1 − ga1 ) maintains the same haplotype across three types of genes, which is a combination of low copy number of ZmGa1Ps-m , non-functional ZmPME3 (barely expressed and lack of complete gene sequence) and ZmPRP3 [ ZmGa1Ps-m-, ZmPME3-, ZmPRP3 + (−+)]. The second evolutionary branch: par2 and mexicana contains high copy numbers of five pollen expressed PME gens, ZmPME3 with potential enzymatic activity, and ZmPRP3 [ ZmGa1Ps-m + , ZmPME3 + , ZmPRP3 + (+++)], which was domesticated to lan 2 [ ZmGa1Ps-m + , ZmPME3 + , ZmPRP3 + (+++)]. An improved population was selected from lan2 proceeded in two directions: one is the loss of ZmPRP3 , forming modern Ga1-S type lines [ ZmGa1Ps-m + , ZmPME3 + , ZmPRP3- (++−)], the other is the loss of ZmPME3 function (caused by a 1 or 2 bp insertion, which is different from the haplotype in ga1 lines), forming modern Ga1-M type lines [ ZmGa1Ps-m + , ZmPME3-, ZmPRP3 + (+−+)] (Fig. 4c and Supplementary Fig. 30 ). Given the huge structural variation at the Ga1 locus, the occurrence of recombination was inhibited and thus the independent variation of the three type of maize was maintained. Unilateral cross incompatibility (UCI) is a fascinating biological phenomenon, related to prezygotic speciation processes, and can offer an effective method of manipulating crosses for crop improvement. Although it was discovered nearly a century ago, we are only now beginning to understand the genetic model and molecular mechanisms underlying this phenomenon. Here, we reported three different types, a total of seven linked genes underlying the Ga1 locus, which control UCI phenotype by affecting pollen tube growth with both antagonistic and synergistic manner. After artificially creating three haplotypes that do not exist in nature [ ZmPME3 OE+ : ZmPME3 + ,ZmPRP3 + (++); CR-Zmprp3 : ZmPME3-, ZmPRP3- (−)], we can now complete a total of eight cross combinations between the three types of genes (Fig. 4d ). The observed phenotypes of these cross combinations matched with the expected phenotype from genotypes across three types of genes. According to previous studies, ga1 pollen tubes accumulate excess levels of highly methylesterified pectins at the apex region when growing through the Ga1-S silk. However, this phenotype does not appear when Ga1-S pollen tubes grow through the Ga1-S silk or ga1 pollen tubes grow through the ga1 silk [14] . This suggest that silk-expressed and pollen-expressed PME genes work together to maintain the balance of pectin esterification/de-esterification at the apical region of the pollen tube cell wall. Our current study provided direct evidence for the existence of two types of PME genes and showed that over-expressed ZmPME3 in the ga1 silk can significantly decrease the degree of methylesterification of silk cell walls and decrease ga1 pollen tube growth rate, providing valuable information about how PME genes regulate UCI. It is possible that (i) ZmPME3 activity accumulates more low-methylesterified pectin, therefore solidifies the silk cell walls and thus establishes a stronger barrier for growing pollen tubes [44] ; (ii) ZmGa1Ps-m inactives ZmPME3 , thereby overcoming the incompatibility effect of ZmPME3 . ZmPRP3 appears to be an accelerator of pollen tube growth in a pathway independent from PME genes, and thereby plays an auxiliary role in the Ga1 genetic model. To date, secreted CRPs have been mainly reported as ligands of receptors or other cell surface proteins, such as LUREs and RALFs in Arabidopsis [45] , [46] , [47] , [48] , and ES1-4 in maize [49] . It thus appears very likely that ZmPRP3 affects pollen tube growth after ligand-receptor binding. The fact that enriched DEGs in maize lines lacking ZmPRP3 were related to metal ion binding suggest that pathways controlled by ZmPRP3 display a high redox potential and may involve ROS metabolism [50] , [51] . Future studies are required to investigate whether a receptor exists in the ga1 pollen tube that interacts with ZmPRP3 , in order to determine the mechanism underlying its pollen tube growth promoting activity. In summary, this study provides important scientific insights into the genetic and molecular basis of UCI and demonstrates its clear evolutionary route, propelling us forward in better understanding reproductive isolation and evolutionary history of modern maize. This knowledge can be used to enhance maize improvement, such as creating artificially isolated varieties for the preservation of important germplasm resources and preventing gene flow from transgenic plants to existing core germplasms in future breeding strategies. Fine mapping of the Ga1 locus A high-density genetic map for the Z58 × SK recombination inbred lines (RIL) population was constructed with 2798 genetic bins [21] via the Illumina MaizeSNP50 BeadChip (Illumina Inc) that contains 56,110 single nucleotide polymorphisms (SNPs), and thus allows to scan the genotype ratio of the two parents in each RIL on the whole genome level. On the basis of Mendel’s model, the expected ratio of the two parents genotype is 1:1. We calculated the actual genotype ratio of for each bin and used the Chi-square Test to assess segregation distortion locus by setting P = 1.79E-06 ( P ≤ 0.05/2798) as the threshold value for segregation distortion significance. 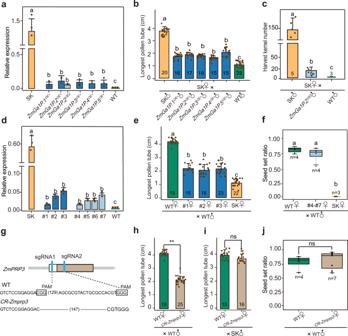Fig. 2: Transgenic confirmation thatZmGa1Ps-m, ZmPME3andZmPRP3regulate pollen tube growth. aQuantitative expression analysis ofZmGa1Ps-mgenes in pollen of over-expressed transgenic plants, WT [KN5585 (ga1)] and SK.bComparison of the longest pollen tubes in SK silks at 8 h after pollination, using pollen of WT, SK, and over-expressed lines for eachZmGa1Ps-mgenes.cStatistical analysis of SK seed set ratio crossed with SK, WT,ZmGa1P.2over expressed lines pollen. dQuantitative expression analysis ofZmPME3in silks ofZmPME3over expressed lines, WT and SK. #1-#3 represents threeZmPME3over expressed transgenic plants. #4-#7 represents fourZmPME3over expressed transgenic plants.eComparison of the longest pollen tubes of WT [KN5585 (ga1)] at 8 h after pollination in silks ofZmPME3over expressed, WT and SK plants.fStatistical analysis of the seed set ratio from crosses by using SK, WT, andZmPME3over expressed plants each as a female parent and WT [KN5585 (ga1)] as a common male parent.gSequence ofZmPRP3in WT and CRISPR-Cas9 edited plants. Lines in blue denote the sgRNA, and the protospacer-adjacent motif (PAM, NGG) is indicated by the black square. White box indicates the coding sequence and barwin is highlighted with brown boxes.hComparison of the longest pollen tubes of WT [KN5585 (ga1)] at 8 h after pollination in silks of WT andCR-Zmprp3plants.iComparison of the longest pollen tubes of SK at 8 h after pollination in silks of WT andCR-Zmprp3plants.jStatistical analysis of seed set ratio from crosses by usingCR-Zmprp3and WT each as a female parent and WT [KN5585 (ga1)] as a common male parent. Fora–f, data were analyzed according to the LSD test. Forh–j, data were analyzed by two-tailed Student’st-test. Error bars represent mean + SD (a–e,h,i). a, b, c indicate significant differences (P< 0.01) (a–f). Asterisks indicate significant differences (**P< 0.01) (h), ns (not significant,P> 0.05) (j). Relative expression (n= 3, biologically independent samples) (a,d). Longest pollen tube length or harvest kernel number (n= number of biologically independent samples in each column) (b,c,e). In box plots, the center line represents the median, box edges delimit lower and upper quartiles and whiskers show the highest and lowest data points, n present sample size (f,j). Source data are provided as a Source Data file. A F 2 mapping population was produced from a cross between SK and Z58, approximately 4900 individuals resulted from the self-pollination of the F 2 plant and were genotyped with molecular markers (see Supplementary Table 2 ) to identify the degree of segregation distortion using the Chi-square test. Molecular marker M1 is cited from Bloom and Holland [24] . M5 and M6 are cited from ref. 22 . Segregation distortion was used as phenotype to narrow down the Ga1 candidate region. Genome-wide association analysis A genome-wide association study (GWAS) of male function of the UCI system was performed using the mixed linear model [52] implemented in the software TASSEL 3.0 [53] that took into account population structure (Q) and familial relationship (K). SNPs with minor allele frequency (MAF ≥ 5%) in the 498 inbred lines from association mapping panel (AMP) were employed in the association analysis. P -value of each SNP were calculated, and significance was defined at a uniform threshold of 8 × 10 −9 ( P = 0.01/ N , N = 1,250,000, Bonferroni correction). The phenotypic value of each inbred lines in the association test was assigned on a 0 to 3 scale (Supplementary Fig. 4 ) to present the degree of cross incompatibility and compatibility when CML304 ( Ga1-S ) was used as female parent and the inbred lines from the AMP were used as male parent. Identification of Ga1-S, Ga1-M and ga1 inbred lines in the AMP CML304 ( Ga1-S ) was used as female parent and inbred lines from the AMP were used as male parents to perform crossing experiments, and the ratio of seed set was used as phenotype to identify inbred lines’ genotypes. When the ratio of seed set was less than 0.1, we identified inbred lines as ga1 types. When Z58 ( ga1 ) was used as male parent, non-ga1 inbred lines were used as female parent, and the ratio of seed set was less than 0.1, we identified inbred lines as Ga1-S types. When the ratio of seed set was greater than 0.5, we identified inbred lines as Ga1-M types. SNP calling and principal component analysis Deep DNA re-sequencing data (~20×) of all 367 lines from the AMP, 68 lines of Zea mays ssp parviglumis (the precursor of modern maize, hereafter named parviglumis ) and 49 lines of Zea mays ssp. mexicana (hereafter named mexicana ], and 336 lines of landraces were first processed using FastQC (v0.11.3) and Trimmomatic (v0.33) to remove poor-quality base calls and adaptors. Reads were then mapped to the B73 and SK reference genome using bowtie2-2.3.3 (with the parameters “–very-fast and–end-to-end”, respectively) [54] . Unique mapped reads were sorted and indexed using Picard (v1.119). SAMtools (v1.3.1) [55] and GATK (v3.5) were used for SNP calling. SNP call was carried out with mapping quality (MQ > 20.0), and thresholds set by sequencing coverage based on minimum coverage (DP > 5) and maximum coverage (DP < 200). Variants from 820 lines were then combined by GATK CombineVariants into a single variant calling file. Finally, sites with a missing rate lower than 25% in all samples were included. Smartpca [56] , [57] was used to perform principle component analysis (PCA) with 130,680 combined SNPs (53,173 SNPs from the B73 reference genome, and 77,507 from the SK reference genome). Calculating reads count, visualization of haplotype clusters Considering the high sequence identity shared among ZmGa1Ps-m genes, we used all reads without filtering unique reads. Read counts of each gene within the Ga1 locus were calculated using subread-1.6.3 tools featureCount s [58] . 141 SNPs (33 SNPs from a 1Kb upstream of ZmPME3 , 58 SNPs within ZmPME3 gene region and 50 SNPs from a 1 Kb downstream of ZmPME3 ) were selected. Haplostrips [59] was used to reveal haplotype clusters in multiple populations. Genomic variation detection A genomic fragment of B73 v4 from chromosome 4: 7 Mb ~ 12 Mb was used as the initial reference genome, a SK genomic fragment derived from chromosome 4: 7 Mb ~12 Mb was aligned to the reference genome with local NCBI-BLAST-2.7.1 [60] following the parameters “-evalue 1e-5 -max_target_seqs 1 -num_threads 10 -perc_identity 95”. 1 kb sequence upstream and downstream of each annotated gene within the Ga1 locus based on SK and B73 genome was collected and aligned to the whole B73 and SK genomes using parameters “-evalue 0.01 -max_target_seqs 1 -num_threads 10 -perc_identity 70” in order to identify homologs. Genomic sequence alignment was displayed using the R package genoplotR [61] , and homologous gene alignment was generated using jcvi [62] . RNA-seq analysis Total RNAs were extracted from pollen and silks of SK, P178 and Z58 using the Quick RNA Isolation Kit (Huayueyang, China). Three technical replicates were performed for each sample. RNA libraries were constructed according to the TruSeq1 Stranded mRNA Sample Preparation Guide (TruSeq1 Stranded mRNA LTSetA). All libraries were PE150 sequenced using an Illumina HiSeq3000 system. Low quality reads were filtered out with Trimmomatic (v0.36) [63] . RSEM-1.3.0 [64] was used to align RNA-seq reads to the B73 v4 and SK reference genome respectively, and gene expression levels were estimated using default parameters. Quantitative RT-PCR and re-sequencing of ZmPME3 and ZmPRP3 Total RNAs were extracted from silks of 70 accessions from the AMP and silks or pollen from transgenic maize plants using the Trizol reagent (Invitrogen). First-strand cDNA was synthesized using EasyScript One-Step gDNA Removal and cDNA Synthesis SuperMix (Transgene Biotech). Real-time fluorescence quantitative PCR with SYBR Green Master Mix (Vazyme Biotech) on a CFX96 Real-Time System was performed to quantify relative expression levels of ZmPRP3 and ZmPME3 . Each set of experiments was repeated three times. The relative quantification method (2 −ΔΔCt ) was used to evaluate quantitative variation. 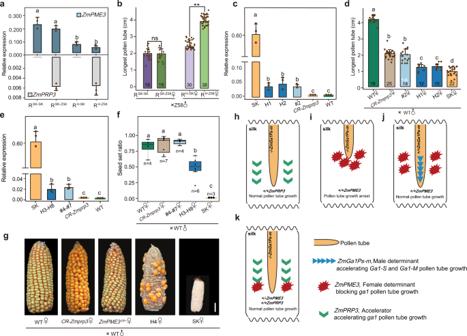Fig. 3: Genetic relationship between three types of genes of theGa1locus. aQuantitative expression analysis ofZmPRP3andZmPME3in silks of RSK-Z58, RSK-SK, RH-Z58, and RH-SK.bComparison of the longest pollen tubes of Z58 at 8 h after pollination in silks of RSK-Z58and RSK-SKsilks, and in RH-Z58and RH-SK.cQuantitative expression analysis ofZmPME3in silks of WT,ZmPME3OE+,CR-Zmprp3, andZmPME3OE+/ CR-Zmprp3. #2 representsZmPME3OE+plant. H1 and H2 represent twoZmPME3OE+/ CR-Zmprp3plants.dComparison of the longest pollen tubes of WT [KN5585 (ga1)] at 8 h after pollination in silks ofCR-Zmprp3,ZmPME3OE+, WT, SK andZmPME3OE+/CR-Zmprp3plants.eQuantitative expression analysis ofZmPME3in silks ofCR-Zmprp3, ZmPME3OE+, WT, SK andZmPME3OE+/CR-Zmprp3plants. H3-H8 represents sixZmPME3OE+/CR-Zmprp3plants. #4-#7 represents fourZmPME3OE+plant.fStatistical analysis of the seed set ratio from crosses by using SK,ZmPME3OE+, CR-Zmagp1,ZmPME3OE+/CR-Zmagp1and WT each as a female parent, WT [KN5585 (ga1)] as a common male parent. H3-H8 represents sixZmPME3OE+/CR-Zmprp3plants. #4-#7 represent fourZmPME3OE+plants.gCrossing experiments showing ears of WT after self-pollination and crosses when SK,ZmPME3OE+, CR-Zmagp1,ZmPME3OE+/CR-Zmagp1were used as female parents, WT [(KN5585,ga1)] pollen was used as male parent. Scale bar = 2 cm.hga1andGa1-Msilk-expressedZmPRP3acts as an accelerator, promoting the growth ofga1pollen tubes.iSilk-expressedZmPME3exists inGa1-Ssilk and is a female determinant that blocksga1pollen tube grow through silk.jZmGa1Ps-mgenes are male determinants, which exist inGa1-SandGa1-Mpollen and can completely overcome block effect ofZmPME3.kWhenZmPME3is heterozygous, introducingZmPRP3can effectively break the block effect ofZmPME3, promotega1pollen tube growth. Fora,c–f, data were analyzed according to the LSD test. Forb, data were analyzed by two-tailed Student’st-test. Error bars represent mean + SD (a–e). a, b, c indicate significant differences (P< 0.01) (a,c–f). Asterisks indicate significant differences (**P< 0.01) (b). ns (not significant,P> 0.05) (b). Relative expression (n= 3, biologically independent samples) (a,c,e). Longest pollen tube length (n= number of biologically independent samples in each column) (b,d). In box plots, the center line represents the median, box edges delimit lower and upper quartiles and whiskers show the highest and lowest data points,npresent sample size (f). Source data are provided as a Source Data file. 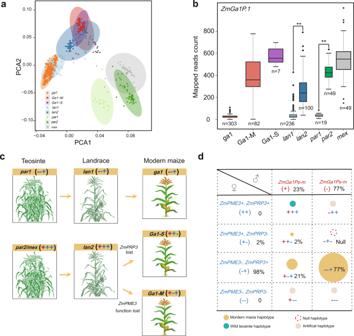Fig. 4: Evolution and modification of theGa1locus during maize domestication. aPrincipal component analysis (PCA) of theGa1locus inparvivglumis,mexicana(mex), landraces,Ga1-M, Ga1-Sandga1inbred lines.bMapped reads count ofZmGa1P.1in the twoparviglumissubgroups (par1, par2),mexicana (mex), two landrace subgroups (lan1, lan2) and modern maize subgroups (Ga1-S, Ga1-Mandga1inbred lines). **P< 0.01 (two-tailed Student’st-test and Wilcoxon ranked sum test). In box plots, the center line represents the median, box edges delimit lower and upper quartiles and whiskers show the highest and lowest data points.npresent sample size. Mapped reads counts are provided in Supplementary Data6.cA putative evolutionary history of theGa1locus during domestication and improvement. The genotype ofZmGa1Ps-mis highlight with red, the genotype ofZmPME3andZmPRP3are highlight with blue. −+ presents a haplotype that lostZmGa1Ps-mandZmPME3(lack of complete gene sequences in the genome) but possessesZmPRP3. +++ presents a haplotype that possessesZmGa1Ps-m,ZmPME3(with potential enzymatic activity) andZmPRP3. ++−presents a haplotype possessesZmGa1Ps-m, functionalZmPME3but lostZmPRP3. +−+presents a haplotype possessesZmGa1Ps-m, ZmPRP3butZmPME3lost their funtion (due to 1 or 2 bp insertion).dEight cross combinations across three types of genes.ZmGa1Ps-mgenes are highly expressed in pollen, the genotype ofZmGa1Ps-mis highlight with red.ZmPME3andZmPRP3are expressed in silk, the genotype ofZmPME3andZmPRP3are highlight with blue. Three haplotypes exist in modern maize inbred lines [ga1:−+;Ga1-S: + + −;Ga1-M: + − + ]. One haplotype exists in wild teosinte [par2/Mexicana: +++]. Null haplotype presents cross incompatibility betweenga1pollen andGa1-Ssilk [ZmGa1Ps-m-, ZmPME3+, ZmPRP3-(−+−)]. Three artificial haplotypes that do not exist in natural collections were:ga1pollen crossed ontoZmPME3over expressed lines [ZmGa1Ps-m-,ZmPME3+, ZmPRP3+ (−++)]Ga1-Spollen crossed ontoZmPRP3knock-out lines [ZmGa1Ps-m+, ZmPME3-, ZmPRP3-(+−)], andga1pollen crossed ontoZmPRP3knock-out lines [ZmGa1Ps-m-, ZmPME3-, ZmPRP3-(−−−)], which all resulted in successful crosses, proving the three artificial haplotypes are fertile. The number labeled in black represent the proportion of male gametes, female gametes and zygote haplotype in AMP. Primers used to re-sequence and quantify expression level of ZmPME3 (in 70 maize inbred lines [15] ) listed in Supplementary Table 3 . Primers that used to amplify and sequence gene regions of ZmPRP3 (in 38 maize inbred lines) are also listed in Supplementary Table 3 . Sequences were aligned with mafft-7.037 [65] , [66] to identify small indels and other variants in the different maize lines. Transgenic validation of ZmPRP3 , ZmGa1Ps-m genes, and ZmPME3 We synthesized a 1261 bp genomic DNA fragment from ZmGa1Ps-m genes (from ATG to TAA, ref to SK) and 1296 bp genomic DNA fragment from ZmPME3 (from ATG to TGA, ref to SK) for the over-expression study. The ZmUbi promoter was inserted into the modified binary vector pCAMBIA3300 to drive gene expression and transformed into the maize inbred line KN5585. We also performed CRISPR-Cas9 based gene editing for four CRP genes. Two ZmPRP3 specific guide-RNAs were incorporated into the pCPB-ZmUbi-hspCas9 vector [39] and targeted ZmPRP3 single exon. Two Zm00001d048948 specific guide-RNAs and two guide-RNAs for targeting Zm00001d048949 and Zm00001d048950 were also incorporated into pCPB-ZmUbi-hspCas9 vectors at once to generate CR-Zm00001d048948 mutant and CR-Zm00001d048949, CR-Zm00001d048950 double mutant respectively. Primers and gene sequence used for transgenic experiments are listed in Supplementary Table 3 . In vivo pollen-tube growth assay All experimental silks were collected at 8 or 24 h after pollination, and fixed in Carnoy’s fluid for 12 h. Fixed silks were washed in a series with the 30%, 50%, 70% cethanol and immersed in 2 M NaOH overnight for tissue softening. Silks were then stained with 0.1% aniline blue (Amresco) for 2 h. Samples were observed under a Nikon ECLIPSE 90i microscope equipped with an ultraviolet filter. Fifteen pollen tubes from at least three plants were examined in each cross. Immunolabeling analysis To visualize the degree of pectin esterification in different silk cells at 8 h after pollination, silks were first fixed in 4% FAA. After dehydration using a 30%, 50%, 70% ethanol series, silks were embedded in paraffin. 2 µm sections were cut from embedded samples and collected on glass slides, and incubated with primary antibody (LM20; LM19, Plant Probes, diluted at 1:20) in a PBS-Tween buffer (1% BSA and 0.05% Tween 20) for 1 h at room temperature. FITC coupled anti-rat IgG (ABclone) was used as a secondary antibody at a 1:500 dilution. Fluorescence signals were recorded with a confocal laser scanning microscope (Zeiss) and measured with ImageJ software [67] . Each image was transformed to an eight-bit image, Next, signal areas were selected with the option “create selection” and measured with the menu tool “measure”. Signal intensity was measured and represented as total fluorescence value divided by the area. 15 silk cells from at least three individual plants were employed for analysis. Statistical analysis Statistical calculations (mean, SD, t -test, LSD test and Wilcoxon ranked sum test) were performed by using Microsoft Excel software and R. Shapiro–Wilk normality test was used to test the normal distribution of each set of data (Supplementary Data 7 ). Statistical significance of differences between sets of data was assessed by using a two-tailed Student’s t -test and Wilcoxon ranked sum non-parametric test. The statistical significance of differences between multiple groups of data was determined by using a LSD test. Differences between two datasets or multiple datasets were considered significant at P < 0.01. Exact P values are provided in Source Data file. Reporting summary Further information on research design is available in the Nature Research Reporting Summary linked to this article.